Two-dimensional quasi-freestanding molecular crystals for high-performance organic field-effect transistors Two-dimensional atomic crystals are extensively studied in recent years due to their exciting physics and device applications. However, a molecular counterpart, with scalable processability and competitive device performance, is still challenging. Here, we demonstrate that high-quality few-layer dioctylbenzothienobenzothiophene molecular crystals can be grown on graphene or boron nitride substrate via van der Waals epitaxy, with precisely controlled thickness down to monolayer, large-area single crystal, low process temperature and patterning capability. The crystalline layers are atomically smooth and effectively decoupled from the substrate due to weak van der Waals interactions, affording a pristine interface for high-performance organic transistors. As a result, monolayer dioctylbenzothienobenzothiophene molecular crystal field-effect transistors on boron nitride show record-high carrier mobility up to 10 cm 2 V −1 s −1 and aggressively scaled saturation voltage ~1 V. Our work unveils an exciting new class of two-dimensional molecular materials for electronic and optoelectronic applications. The research on two-dimensional (2D) layered materials has been thriving for a decade now since the discovery of graphene [1] , [2] , [3] . Most of the 2D materials studied so far, including graphene, chalcogenides and oxides, are inorganic atomic crystals with strong in-plane chemical bonds [3] . 2D molecular crystals held by van der Waals (vdW) forces, on the other hand, are rarely reported. Organic molecular crystals represent an important class of materials for electronic and photonic applications [4] , [5] , [6] , [7] . Compared with bulk materials, monolayers could effectively eliminate interlayer screening, thus offer an ideal system to directly probe the effect of disorders [8] , [9] and interfaces [10] , [11] on charge transport. Furthermore, both carrier injection and modulation would become more efficient to greatly improve the performance of organic field-effect transistors (OFETs). Therefore, 2D molecular crystals can open a new paradigm in the applications of layered materials and heterostructures. Here, we report on the epitaxial growth and OFETs of 2D dioctylbenzothienobenzothiophene (C 8 -BTBT) molecular crystals down to monolayer on graphene and hexagonal boron nitride (abbreviated as BN) substrates. We select C 8 -BTBT because it is among the highest mobility small-molecule organic materials [12] , [13] , [14] . Graphene and BN are also ideal substrates as they are atomically flat without dangling bonds [15] . Therefore, the initial stage of epitaxy relies on the vdW interaction between the molecules and substrate [16] . We show that the substrate flatness and weak vdW interaction are crucial for high-performance monolayer organic transistors because of the minimal disturbance in both crystal growth and charge transport. Growth and characterization of C 8 -BTBT molecular crystals The growth was carried out in a tube furnace under high vacuum of ~4 × 10 −6 Torr without carrier gas ( Supplementary Fig. 1 ). We heated up the C 8 -BTBT powder (as received from NIPPON KAYAKU Co., Ltd. without further purification) to 100–120 °C and placed graphene or BN on SiO 2 /Si a few inches away from the source to start the growth. Below we focus our discussion on graphene substrate, while similar observations are also made on BN ( Supplementary Figs 2 and 3 ). Figure. 1b–e show sequential atomic force microscopy (AFM) snapshots of the same sample during a 95-min growth, which was intentionally interrupted for characterization (the sample was taken out to ambient each time, see Supplementary Fig. 4 for the AFM images of the whole sequence). From these images, several conclusions can be drawn. (i) The crystals preferentially grew on graphene, in a layer-by-layer fashion with atomic smoothness. The thickness of the initial two layers (namely the interfacial layer, IL, and the first layer, 1L) was ~0.6 nm and ~1.7 nm, respectively ( Fig. 1f , Supplementary Fig. 5 ), indicating that molecular packing in the initial layers was different from bulk crystals [12] . However, the thickness of the subsequent layers was ~3 nm as bulk crystals. (ii) In each layer, the growth initiated at certain nucleation sites and proceeded nearly isotropically as compact islands. The most common nucleation sites were disorders from the previous layers ( Fig. 1c ) or from the substrate ( Fig. 1d , Supplementary Fig. 4a,f,m ), as well as edges ( Fig. 1e , Supplementary Fig. 4k,n ), likely due to their high surface energy. (iii) The frequent interruption and ambient exposure of the sample did not significantly affect the growth, which suggested that the crystals were of pristine quality and stable against photooxidation in ambient. Supplementary Figure 6 shows the growth process of another sample with excellent quality and thickness control. 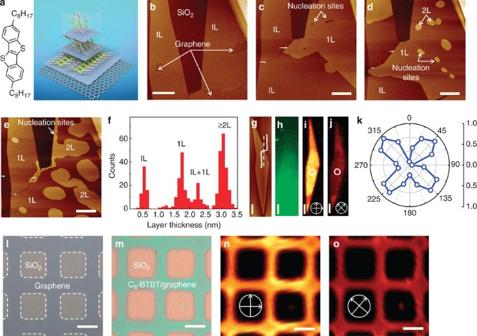Figure 1: Epitaxial growth of C8-BTBT molecular crystals on graphene. (a) Cartoon illustration of the molecular structure of C8-BTBT (left panel) and their packing on graphene (right panel). (b–e) Sequential AFM snapshots of a sample at different stages during a 95-min growth. Scale bar, 2 μm. The complete sequence of the growth process is shown inSupplementary Fig. 4. (f) Histogram of layer thickness of C8-BTBT molecular crystals on graphene, taken from over 10 samples. (g–j) AFM (g), Raman mapping (h) and cross-polarized optical micrographs (i,j) of a uniform 1L C8-BTBT crystal grown on graphene. Scale bar, 3 μm. Inset ofgis the height profile along the dashed line. The total thickness of graphene and the crystal is 3.7 nm, confirming 1L C8-BTBT (2L would have made the total thickness greater than 5.3 nm). The Raman spectrum of the C8-BTBT crystal is plotted inSupplementary Fig. 13b. (k) Normalized intensity of the 1L C8-BTBT crystal under cross-polarized optical microscope as a function of rotation angle. The data are taken at the marked spot iniandj. (l–o) Patterned growth of C8-BTBT crystal on graphene. Scale bar, 7 μm. (l,m) Optical microscopy image of a plasma-patterned graphene before and after C8-BTBT growth, respectively. (n,o) Cross-polarized optical micrographs of the same area after C8-BTBT growth. The uniform colour change over the entire area confirms that C8-BTBT forms a single crystal. Figure 1: Epitaxial growth of C 8 -BTBT molecular crystals on graphene. ( a ) Cartoon illustration of the molecular structure of C 8 -BTBT (left panel) and their packing on graphene (right panel). ( b – e ) Sequential AFM snapshots of a sample at different stages during a 95-min growth. Scale bar, 2 μm. The complete sequence of the growth process is shown in Supplementary Fig. 4 . ( f ) Histogram of layer thickness of C 8 -BTBT molecular crystals on graphene, taken from over 10 samples. ( g – j ) AFM ( g ), Raman mapping ( h ) and cross-polarized optical micrographs ( i , j ) of a uniform 1L C 8 -BTBT crystal grown on graphene. Scale bar, 3 μm. Inset of g is the height profile along the dashed line. The total thickness of graphene and the crystal is 3.7 nm, confirming 1L C 8 -BTBT (2L would have made the total thickness greater than 5.3 nm). The Raman spectrum of the C 8 -BTBT crystal is plotted in Supplementary Fig. 13b . ( k ) Normalized intensity of the 1L C 8 -BTBT crystal under cross-polarized optical microscope as a function of rotation angle. The data are taken at the marked spot in i and j . ( l – o ) Patterned growth of C 8 -BTBT crystal on graphene. Scale bar, 7 μm. ( l , m ) Optical microscopy image of a plasma-patterned graphene before and after C 8 -BTBT growth, respectively. ( n , o ) Cross-polarized optical micrographs of the same area after C 8 -BTBT growth. The uniform colour change over the entire area confirms that C 8 -BTBT forms a single crystal. Full size image The sample in Fig. 1b–e has multiple nucleation sites in each layer, probably due to the defects such as cracks and wrinkles of the underlying graphene ( Supplementary Fig. 4a ). However, with careful control of the growth parameters on defect-free graphene, we repeatedly observed large-area uniform 1L or 2L C 8 -BTBT single crystals up to ~80 μm in size ( Supplementary Figs 7–11 . Figure 1g shows a uniform monolayer C 8 -BTBT crystal grown on a graphene sample over 30 μm long and 5 μm wide (we do not count the IL in the number of layers because charge transport does not likely happen in this layer, as discussed later), as confirmed by the total thickness of 3.7 nm ( Fig. 1g inset) and Raman spectroscopy ( Fig. 1h , Supplementary Fig. 13b ). Cross-polarized optical micrographs showed that the entire piece was a single crystal except a small portion at the bottom ( Fig. 1i,j ), and the optical intensity had a fourfold symmetry as expected for high-quality single crystal ( Fig. 1k ). The low nucleation density and island growth mode (as opposed to fractal growth) point to a high diffusion coefficient of C 8 -BTBT molecules both on surface and along the island edges [17] , [18] . This is a natural result of the substrate flatness ( Supplementary Fig. 12 ) and relatively weak vdW forces from the substrate, in clear contrast to the conventional epitaxy where strong chemical bonds are formed at the interface [16] . The thickness of ~0.6 nm for the IL pointed to a new form of molecular packing at the interface. To determine its structure, we performed combined scanning tunnelling microscopy (STM) and density functional theory (DFT) studies (see Methods for details). We observed under STM that the IL C 8 -BTBT molecules were packed in a rectangular lattice with d 1 =2.52 nm and d 2 =0.66 nm in two orthogonal directions ( Fig. 2a ). On the basis of this morphology, we built a series of possible molecular configurations, where the C 8 -BTBT molecule unit was leaning towards graphene by different angles compared with the ‘stand-up’ configuration ( Supplementary Fig. 14 ). We found that the most stable single-molecule configuration had a leaning angle of ~35°, in which both alkyl chains and benzothiophene were in closest proximity and parallel to graphene ( Supplementary Fig. 14f ). In such configuration, both CH-π interactions [19] and the π–π interactions [20] were maximized. When forming periodic crystals, however, the fully relaxed benzothiophene plane was slightly tilted to form a 10° angle with graphene in DFT, due to intermolecular interactions. We further calculated the stability as a function of lattice constants and found that d 1 =2.47 nm and d 2 =0.64 nm was the most stable configuration ( Supplementary Fig. 15 ), in excellent agreement with STM results. Moreover, the angle between the carbon chains and the benzothiophene was calculated to be 134°, very close to the measured angle of 140° by STM. Finally, quantitative match with both the layer thickness ~0.52 nm and detailed STM height profiles ( Supplementary Fig. 23 ) allowed us to confirm the crystal structure of the IL drawn in Fig. 2b . Clearly, the symmetry of IL is different from that of the underlying graphene substrate because of the vdW nature of the epitaxy [16] . Our DFT calculations suggest that 2D growth of IL is energetically favourable due to the intermolecular interactions ( Supplementary Figs 16–18 , Supplementary Note 1 ). In addition, a global energy minimum exists for different IL orientations with respect to the graphene substrate ( Supplementary Fig. 19 , Supplementary Note 2 ), making it possible to form large-area single crystals as observed experimentally ( Supplementary Fig. 10 ). We note that IL does not likely contribute to lateral charge transport due to small intermolecular π–π interactions. 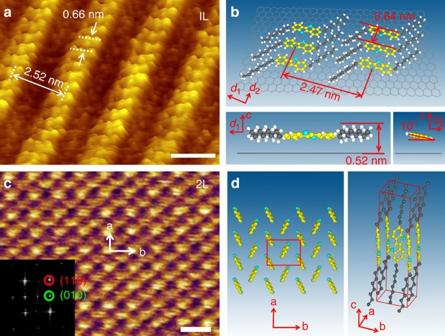Figure 2: Molecular structure of the C8-BTBT crystals on graphene. (a) A constant-current STM image of the IL on CVD graphene (Vsample=−0.91 V andI=12.9 pA). Scale bar, 2 nm. (b) Top view (top panel) and side view (bottom panels) of the most stable IL structure obtained by DFT calculations. The lattice constants of 2.47 nm and 0.64 nm are in excellent agreement with experiments. (c) High-resolution AFM image of the 2L on graphene. The unit cell is marked. Inset is the Fast Fourier Transform of the AFM image with lattice indices. Scale bar, 1 nm. (d) Top view (left panel) and side view (right panel) of the 2L structure according to the AFM image inc. Figure 2: Molecular structure of the C 8 -BTBT crystals on graphene. ( a ) A constant-current STM image of the IL on CVD graphene ( V sample =−0.91 V and I =12.9 pA). Scale bar, 2 nm. ( b ) Top view (top panel) and side view (bottom panels) of the most stable IL structure obtained by DFT calculations. The lattice constants of 2.47 nm and 0.64 nm are in excellent agreement with experiments. ( c ) High-resolution AFM image of the 2L on graphene. The unit cell is marked. Inset is the Fast Fourier Transform of the AFM image with lattice indices. Scale bar, 1 nm. ( d ) Top view (left panel) and side view (right panel) of the 2L structure according to the AFM image in c . Full size image Due to limited vertical conductivity, the structure of the subsequent layers was studied by high-resolution AFM. We found that the crystal structures for both 1L and 2L were monolithic with herringbone-type packing as in bulk crystals [12] ( Fig. 2c , d , Supplementary Figs 9–11 , 24 ). The lattice constants were a=6.24±0.25 Å (6.69±0.13 Å), b=8.31±0.05 Å (7.89±0.25 Å) for C 8 -BTBT crystals on graphene (BN), each measured from 10 areas on different samples. The slight deviation from bulk crystal values was not understood, but could come from limited lateral resolution of AFM. We did not observe any statistical difference of lattice constants between 1L and 2L. The C 8 -BTBT molecules in 1L seemed more inclined than bulk crystals [12] . Apparently, the role of substrate was much reduced in 1L and became negligible in 2L and above, because the vdW forces decayed rapidly as r −6 . Indeed, the calculated binding energy of 1L and graphene is 0.07 eV per molecule ( Supplementary Fig. 20 ), much smaller than that of IL as well as intermolecular binding energy within 1L. Importantly, the charge transport in graphene is not significantly affected by the deposition of C 8 -BTBT layers ( Supplementary Fig. 25 , Supplementary Table 1 ). Considering the charge transport in organic transistors occurs near the semiconductor-dielectric interface [11] , [21] , the few-layer C 8 -BTBT crystals can thus be regarded as quasi-freestanding with minimal disturbance from the substrate. For future device applications, it is important to demonstrate the growth of 2D molecular crystals on centimetre scale as well as patterning capability. We successfully grew large-area C 8 -BTBT crystals on graphene formed by chemical vapour deposition (CVD graphene; ~1 cm in size, see Methods for CVD sample preparation), with over 90% coverage ( Supplementary Figs 26–28 , Supplementary Note 4 ). AFM analysis indicated that the C 8 -BTBT crystals on CVD graphene shared the same molecular packing as those on exfoliated graphene. However, due to the polycrystalline nature of the CVD graphene, and the presence of wrinkles, cracks and polymer residue, the C 8 -BTBT films were polycrystalline with domain size around tens of micrometres ( Supplementary Fig. 28 ). Future works are needed to further improve the quality and uniformity of C 8 -BTBT crystals on CVD graphene. Our approach also enables patterning of ultrathin organic crystals for device integration. Figure 1m shows that C 8 -BTBT crystal can be readily grown on graphene patterns etched by oxygen plasma, with excellent uniformity. Cross-polarized optical micrographs verified that the whole area was a single crystal ( Fig. 1n,o ). FETs of 2D C 8 -BTBT crystals Next we demonstrate several logic device applications of the epitaxial C 8 -BTBT crystals. When grown on graphene, a vertical graphene-semiconductor heterostructure was readily obtained. We then deposited 100 nm thick Au layer as top electrode to form a vertical OFET ( Fig. 3b inset). Compared with previously reported 2D layered heterostructures [22] , [23] , [24] , our method is inherently scalable without the need for mechanical transfer. 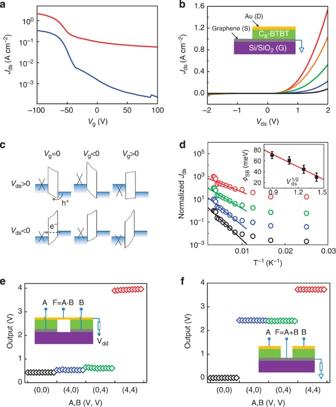Figure 3: Vertical OFETs based on graphene-C8-BTBT heterostructures. (a) Room temperatureJds−Vgcharacteristics of a device with ~15 nm thick (5-layer) C8-BTBT. From top to bottom,Vds=2 V and 1 V, respectively. (b) Room temperatureJds−Vdscharacteristics of the same device ina. From top to bottom,Vg=−100 V, −90 V, −80 V, −70 V and 0 V, respectively. Inset shows the device schematics. The source (S), drain (D) and gate (G) terminals are marked. (c) Energy band diagrams of the vertical OFET under various bias conditions. The band diagram underVds=0 andVg=0 is plotted inSupplementary Fig. 29. (d) Arrhenius plot (symbols) of normalizedJdsof the same device inaunderVg=−100 V. From top to bottom,Vds=2 V, 1.6 V, 1.2 V and 0.8 V, respectively. The plot clearly shows two regimes: thermionic emission at high temperatures and tunnelling at low temperatures. Lines are theoretical fittings of the thermionic emission current. The extractedΦSBare plotted in the inset as a function ofVds1/2(symbols), with a linear fitting (line). (e,f) Output voltage levels of an AND (e) and OR (f) gate comprised two vertical diodes. The insets show the circuit diagrams. The pull-up resistor for the AND gate and the pull-down resistor for the OR gate are both 5 × 109Ohms. During the operation of both logic gates,Vg=−100 V,Vdd=4 V. Figure 3a,b show transfer ( J ds − V g ) and output ( J ds − V ds ) characteristics of a typical vertical FET comprising of five layers of C 8 -BTBT, with a large on/off ratio ~1,500 at room temperature. The device exhibited small but finite hysteresis ( Supplementary Fig. 30 ), likely due to the ambient molecules trapped at the C 8 -BTBT/Au interface. The hysteresis could be minimized by optimizing the deposition process of the top electrode. Another device with thicker C 8 -BTBT showed on/off ratio ~10 6 at room temperature ( Supplementary Fig. 31 ). The devices exhibited diode-like rectifying behaviour similar to graphene barristors [25] , [26] , indicating different conduction mechanisms for the two bias polarities. Considering the energy of the highest occupied molecular orbital (HOMO) and lowest unoccupied molecular orbital (LUMO) of C 8 -BTBT was 5.39 eV and 1.55 eV, respectively [27] , the band diagrams under various bias conditions were drawn in Fig. 3c . Under forward bias, the charge transport was thermionic emission as reflected by the Arrhenius plot in the high temperature regime ( Fig. 3d ). In this regime, holes were thermally activated over a Schottky barrier Φ SB at the metal–semiconductor interface. Φ SB was found to decrease linearly with V ds 1/2 ( Fig. 3d inset) due to the image force as in conventional Schottky junctions [28] . The extrapolated Φ SB at zero V ds was ~140 meV, consistent with the work function of Au. As we changed the Fermi energy of graphene by sweeping V g , the barrier width was altered to realize transistor switching ( Fig. 3c ) as in the case of Schottky-type carbon nanotube transistors [29] . The ultralow leakage current at the off state suggested the absence of pinholes in the crystal even on the graphene edges. Under reverse bias, the thermionic emission current became exponentially small, and the charge transport was dominated by tunnelling through the C 8 -BTBT layers. This was confirmed by the current insensitivity to temperature ( Fig. 3b , Supplementary Fig. 31a–c ) as expected for tunnelling mechanism [22] . The tunnelling current is very small because the orientation of the C 8 -BTBT molecules does not favour vertical charge transport. Therefore the vertical transistors are suitable for low-power applications. Figure 3: Vertical OFETs based on graphene-C 8 -BTBT heterostructures. ( a ) Room temperature J ds −V g characteristics of a device with ~15 nm thick (5-layer) C 8 -BTBT. From top to bottom, V ds =2 V and 1 V, respectively. ( b ) Room temperature J ds −V ds characteristics of the same device in a . From top to bottom, V g =−100 V, −90 V, −80 V, −70 V and 0 V, respectively. Inset shows the device schematics. The source (S), drain (D) and gate (G) terminals are marked. ( c ) Energy band diagrams of the vertical OFET under various bias conditions. The band diagram under V ds =0 and V g =0 is plotted in Supplementary Fig. 29 . ( d ) Arrhenius plot (symbols) of normalized J ds of the same device in a under V g =−100 V. From top to bottom, V ds =2 V, 1.6 V, 1.2 V and 0.8 V, respectively. The plot clearly shows two regimes: thermionic emission at high temperatures and tunnelling at low temperatures. Lines are theoretical fittings of the thermionic emission current. The extracted Φ SB are plotted in the inset as a function of V ds 1/2 (symbols), with a linear fitting (line). ( e , f ) Output voltage levels of an AND ( e ) and OR ( f ) gate comprised two vertical diodes. The insets show the circuit diagrams. The pull-up resistor for the AND gate and the pull-down resistor for the OR gate are both 5 × 10 9 Ohms. During the operation of both logic gates, V g =−100 V, V dd =4 V. Full size image We further demonstrated logic gates by integrating two vertical OFETs. For AND gate, we grew C 8 -BTBT crystals on two adjacent graphene as inputs, and connected them using a common top electrode as output ( Fig. 3e inset). Either diode under forward bias (with a low input) would be closed with a much lower resistance than the pull-up resistor, therefore creating a low output. The gate showed excellent logic function, with the high and low output close to V dd and 0, respectively ( Fig. 3e ). For OR gate, two top electrodes as inputs were deposited on C 8 -BTBT crystal grown on a single graphene as output ( Fig. 3f inset). Either diode under forward bias (with a high input) would be closed with a much lower resistance than the pull-down resistor, therefore create a high output. The non-ideal output for (4, 0) and (0, 4) was due to the finite leakage current under reverse bias ( Fig. 3f ). More complex functionality can be realized with lithographic patterning. Finally, we fabricated planar OFETs with 1L C 8 -BTBT crystals grown on insulating BN ( Fig. 4 , Supplementary Figs 32 and 33 ). Despite the monolayer thickness (~1.7 nm), the devices exhibited several features of ideal OFETs: linear I ds − V g ( I ds 1/2 − V g ) characteristics in the linear (saturation) regime, linear I ds − V ds characteristics at low bias, and negligible hysteresis [4] . The room temperature peak field-effect mobility μ could reach up to ~10 cm 2 V −1 s −1 ( Fig. 4c ), much higher than previously reported values for monolayer OFETs (in the range of ~10 −6 −0.1 cm 2 V −1 s −1 ; refs 30 , 31 , 32 , 33 , 34 ). Note that μ was underestimated due to contact resistance. Interestingly, μ was found to decrease after reaching a plateau as the carrier density gradually increased ( Fig. 4c , Supplementary Fig. 33a ) due to additional sources of scattering such as electron–electron interactions [35] . The drastic improvement of mobility indicated that the density of charge traps and grain boundaries was significantly reduced [8] . This was attributed to the pristine, ultrasmooth crystals and their weak coupling with the substrate, analogous to the case of graphene on BN [15] . The mobility was found to decrease slightly at low temperature in some of our devices ( Supplementary Fig. 33c ). The weak insulating behaviour pointed to finite density of charge traps [9] , [11] , which will be carefully analysed and improved in future works. The performance of monolayer C 8 -BTBT FETs was comparable to 2D atomic crystals such as MoS 2 (refs 36 , 37 , 38 , 39 ), but with a clear advantage of much lower synthesis temperature. 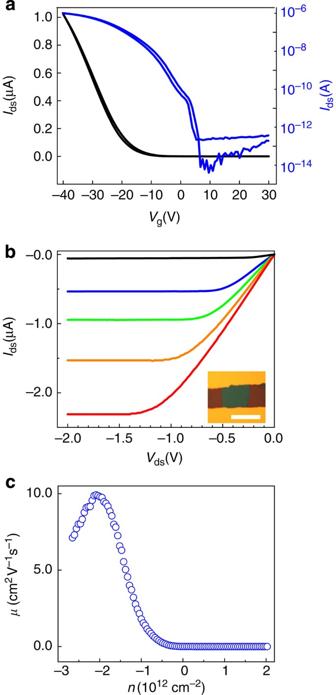Figure 4: Planar OFET of monolayer C8-BTBT molecular crystals on BN. (a) Room temperature double-sweepIds−Vgcharacteristics (Vds=−0.5 V), with little hysteresis. Black and blue lines are drawn in linear and log scales, respectively. (b)Ids−Vdscharacteristics of the device ina. From top to bottom,Vg=−10 V, −25 V, −30 V, −35 V and −40 V, respectively. Inset shows the optical microscopy image of the device. Scale bar, 16 μm. (c) The extractedμ−Vgrelationship at room temperature. The peak mobility is over 10 cm2V−1s−1for this device. Figure 4: Planar OFET of monolayer C 8 -BTBT molecular crystals on BN. ( a ) Room temperature double-sweep I ds −V g characteristics ( V ds =−0.5 V), with little hysteresis. Black and blue lines are drawn in linear and log scales, respectively. ( b ) I ds −V ds characteristics of the device in a . From top to bottom, V g =−10 V, −25 V, −30 V, −35 V and −40 V, respectively. Inset shows the optical microscopy image of the device. Scale bar, 16 μm. ( c ) The extracted μ − V g relationship at room temperature. The peak mobility is over 10 cm 2 V −1 s −1 for this device. Full size image Compared with bulk crystal devices [12] , [13] , [14] , [40] , the I ds − V ds characteristics in Fig. 4b exhibited two unique features: the absence of non-linearity at low bias and a complete saturation with extremely small saturation voltage (~1 V). Both features were direct consequence of the monolayer nature of the channel. The former appeared because the source/drain electrodes were in direct contact with the charge transport layer, leading to extremely efficient carrier injection. The latter was due to easy and complete channel pinch-off without interlayer screening effects [41] . With scaled dielectric thickness and other optimized device parameters, the operation voltage of these OFETs can be reduced to 1 V, which makes these devices compatible with silicon CMOS in circuit applications. In conclusion, we demonstrate that vdW epitaxy on 2D materials provides a viable approach to grow few-layer organic molecular crystals with pristine quality, monolayer thickness control and large-area processability for high-performance and low-cost logic device applications. Compared with the previous efforts to grow organic crystals on 2D materials [26] , [40] , [42] , our results truly demonstrate the advantage of this concept by proving the high quality of the interface. Sample preparation and growth process of C 8 -BTBT crystals We exfoliated graphene and BN on 285 nm SiO 2 /Si as growth substrate without further thermal treatment. The graphene substrates used in this work were monolayer unless otherwise stated. The graphene and BN were characterized by optical microscope, AFM and Raman spectroscopy before growth to obtain the thickness and topological information. For CVD graphene, we first grew the graphene on copper foils (Alfa Aesar) at 1,050 °C under 4 sccm CH 4 and 200 sccm H 2 . With poly(methyl methacrylate) as a support layer, we transferred a 1 cm × 1 cm CVD graphene on to SiO 2 /Si substrate, followed by a thermal annealing at 300 °C in forming gas. The growth of C 8 -BTBT crystals was carried out in a home-built tube furnace. We put the source and sample in the quartz tube and used a turbo molecular pump to evacuate the quartz tube to ~4 × 10 −6 Torr ( Supplementary Fig. 1 ). The distance between source and sample was accurately measured each time to attain good reproducibility. We then heated up the C 8 -BTBT crystal to 100–120 °C to start the growth. In our experiment, the growth of C 8 -BTBT layers was mainly controlled by the source temperature and growth time. To achieve precise control of IL, 1L and 2L growth (for example, the samples in Fig. 1 and Supplementary Figs 5–8 ), the source temperature was 100 °C. The growth time to achieve uniform IL and 1L was approximately 15 and 30 min, respectively, but was sample dependent. For thicker C 8 -BTBT layers (for example, the samples in Fig. 3 ), the source temperature was 120 °C. To terminate the growth, we turned off the furnace and let the sample cool down to room temperature under high vacuum. Characterization of the C 8 -BTBT crystals Two types of AFM were performed in this work. For high-resolution AFM, the experiments were performed on an Asylum Cypher under ambient conditions with Asylum ARROW UHF AFM tips. To get sub-nanometre resolution, samples had to be ultra-flat. So we grew C 8 -BTBT crystals on thick graphite and BN for high-resolution AFM. In this case, the roughness of the substrate did not affect the sample. We did not observe any difference in C 8 -BTBT crystals grown on thick graphite and graphene in terms of the thickness and growth mode of each layer. For regular AFM, the experiments were performed on a Veeco Multimode 8 under ambient conditions. Raman spectroscopy and mapping were performed on a WITec Alpha 300R confocal Raman system with a 532 nm laser excitation (spot size ~300 nm, laser power 1 mW). Cross-polarized optical microscopy was performed on the same WITec Alpha 300R Raman microscope with white light illumination and × 50 objective. During the experiments, the laser notch filter was taken out and two cross-polarized linear polarizers were installed, one between illumination source and sample, the other between sample and detector. The images were acquired by scanning the sample. We integrated the spectrum from 520 to 550 nm to plot the images. The STM study was carried out in a UNISOKU ultrahigh vacuum four-probe SPM. All STM measurements were performed at liquid-nitrogen temperature and the images were taken in a constant-current scanning mode. The STM tips were obtained by chemical etching from a wire of Pt (80%) Ir (20%) alloys. Lateral dimensions observed in the STM images were calibrated using a standard graphene lattice. For better substrate conductivity, the STM samples were prepared on monolayer CVD graphene grown on Cu foils. The samples were overall very flat with small corrugated areas and with some steps on the copper surface ( Supplementary Figs 21 and 22 ). Since high-resolution STM scans were usually recorded in small areas ~100 nm 2 , the substrate roughness was very small and does not affect the STM measurement. Details of DFT calculations The DFT calculations were carried out within the framework of plane-wave DFT, implemented in the Vienna ab initio simulation package [43] . We employed the projector-augmented-wave potentials [44] to describe the electron–ion interaction and the Perdew–Burke–Ernzerhof generalized gradient approximation (PBE-GGA) for exchange-correlation functional [45] . The effect of vdW interactions was described using the semiempirical correction scheme of Grimme, DFT-D2 (ref. 46 ). The kinetic energy cutoff of 400 eV was adopted for the plane-wave expansion and the Brillouin zone was sampled by the Monkhorst–Pack scheme. All atomic positions were fully optimized until the maximum Hellmann–Feynman forces acting on each atom was less than 0.02 eV Å −1 . Fabrication process of OFETs For the vertical OFETs in Fig. 3 , we started by exfoliating monolayer graphene on 285 nm SiO 2 /Si. We transferred a 100 nm thick Au electrode to contact part of the graphene as probing pad before growth of C 8 -BTBT crystals. Briefly, we pre-deposited 100 nm Au film on a glass slide. Then we used a tungsten probe tip attached to a micro manipulator to carefully pick up the Au film and transfer to the target location under microscope [47] . AFM was performed before and after growth to extract the thickness of the crystals. After growth of the crystal, another Au film was transferred as top electrode, which partly overlapped with graphene (but not with the bottom Au electrode). We used mechanical transfer to deposit the Au electrodes to avoid any residue introduced by lithography and any damage of the ultrathin C 8 -BTBT layers by vacuum deposition. Other than the growth, all other fabrication processes were carried out under ambient condition. For the vertical OR gate, the fabrication was similar except that after growth, two separate Au films were used as inputs. The lateral separation between the Au electrodes (tens of micrometers) was three orders of magnitude larger than the separation between Au and bottom graphene (tens of nanometres), therefore the lateral charge transport was negligible. For the vertical AND gate, two adjacent monolayer graphene samples were identified after exfoliation. We transferred two Au electrodes, each contacting one of the graphene samples as probing pads. After growth, an Au film was transferred to overlap both graphene as common top electrode (but not with the bottom Au electrodes). For the planar OFET in Fig. 4 , we first exfoliated BN (with thickness normally <10 nm) on 285 nm SiO 2 /Si substrate. The growth of monolayer C 8 -BTBT crystal was carefully done by heating the source to 120 °C. AFM was performed before and after growth to extract the thickness of the crystals. Finally, two Au films were transferred on the top of the C 8 -BTBT crystal as source and drain electrodes. Electrical measurements of FETs Electrical measurements were carried out by an Agilent B1500 semiconductor parameter analyser in a close-cycle cryogenic probe station with base pressure ~10 −5 Torr. The vertical transistors were annealed in vacuum at 120 °C before measurement to improve contacts, while the planar transistors did not need any annealing step. How to cite this article: He, D. et al . Two-dimensional quasi-freestanding molecular crystals for high-performance organic field-effect transistors. Nat. Commun. 5:5162 doi: 10.1038/ncomms6162 (2014).